Rediscovering black phosphorus as an anisotropic layered material for optoelectronics and electronics Graphene and transition metal dichalcogenides (TMDCs) are the two major types of layered materials under intensive investigation. However, the zero-bandgap nature of graphene and the relatively low mobility in TMDCs limit their applications. Here we reintroduce black phosphorus (BP), the most stable allotrope of phosphorus with strong intrinsic in-plane anisotropy, to the layered-material family. For 15-nm-thick BP, we measure a Hall mobility of 1,000 and 600 cm 2 V −1 s −1 for holes along the light ( x ) and heavy ( y ) effective mass directions at 120 K. BP thin films also exhibit large and anisotropic in-plane optical conductivity from 2 to 5 μm. Field-effect transistors using 5 nm BP along x direction exhibit an on–off current ratio exceeding 10 5 , a field-effect mobility of 205 cm 2 V −1 s −1 , and good current saturation characteristics all at room temperature. BP shows great potential for thin-film electronics, infrared optoelectronics and novel devices in which anisotropic properties are desirable. Current research in layered materials primarily focuses on graphene [1] , [2] , [3] , [4] , [5] , [6] , [7] , [8] , [9] , [10] , insulating hexagonal boron nitride [11] , [12] , [13] , and members from the transition metal dichalcogenides (TMDCs) [14] , [15] , [16] , [17] , [18] , [19] , [20] , [21] family, such as molybdenum disulphide (MoS 2 ) and tungsten diselenide (WSe 2 ). Graphene transistors suffer from a low on–off current ratio because of its zero-bandgap nature. Although transistors made from few-layer TMDCs, such as MoS 2 and WSe 2 , show very high on–off current ratios and excellent current saturation characteristics, the carrier mobility in these TMDCs is much lower than in graphene and fluctuates significantly from less than 10 to around 200 cm 2 V −1 s −1 (refs 21 , 22 , 23 ), restricting their application in both electronics and optoelectronics. Most of the TMDCs currently being studied have band gaps larger than 1 eV, rendering them unsuitable for near-infrared optical telecommunications and mid-infrared applications. Furthermore, in these materials, the photonic, electronic and mechanical properties within the plane of the layers are largely isotropic and do not exhibit a significant directional dependence. In this work, we reintroduce black phosphorus (BP) to the layered-material family as an anisotropic material for optoelectronic and electronic applications. Narrow gap BP thin film (0.3 eV in bulk) can fill the space between zero-gap graphene and large-gap TMDCs, making it an ideal material for near and mid-infrared optoelectronics. BP thin films with a thickness of 15 nm show high mobility above 650 cm 2 V −1 s −1 at room temperature and above 1,000 cm 2 V −1 s −1 at 120 K along the light effective mass ( x ) direction, implying its promising future for high frequency, thin-film electronics. Furthermore, the anisotropic nature within the plane of the layers may allow for the realization of novel thin-film infrared polarizers, infrared polarization sensors, new types of plasmonic devices [24] , phonon transport engineering that can take advantage of the directional dependence of its phonon dispersion and the utilization of the lower effective-carrier-mass along x direction to build high-performance transistors [25] , [26] , [27] . Characterization of BP thin-film layer number Similar to graphite, bulk BP is an elemental layered material. Bulk BP crystal has been studied extensively decades ago and it is the most stable allotrope of phosphorus [28] , [29] , [30] , [31] , [32] because of its unique orthorhombic crystal structure as shown in Fig. 1a . As carbon atoms in graphene, each phosphorus atom is connected to three adjacent phosphorus atoms in BP to form a stable, linked ring structure, with each ring consisting of six phosphorus atoms. However, the puckered BP structure has reduced symmetry compared with graphite, resulting in its unique angle-dependent in-plane conductivities [33] , [34] , [35] , [36] . The adjacent layer spacing is around 0.53 nm and the lattice constant in this orthorhombic system along the z direction is 1.05 nm. Moreover, as in TMDCs, the bandgap in BP is expected to be strongly dependent on the layer number [37] because of the layer–layer coupling. Single or few-layer BP can have very different bandstructures compared with its thin film or bulk form. Recent theoretical investigations reveal that for single-layer BP, the single particle band gap can be as large as 2 eV [38] , [39] . If electron-hole interaction is taken into account, the bandgap can be significantly smaller because of large exciton-binding energy. Furthermore, single and few-layer BP also exhibit strong in-plane anisotropy as in bulk BP. As a result, future exploration on atomically thin BP may lead to new two-dimensional (2D) materials very different from graphene and transition metal dichalcogenides. Recently, the dependence of its band structure on strain was also investigated theoretically [40] . 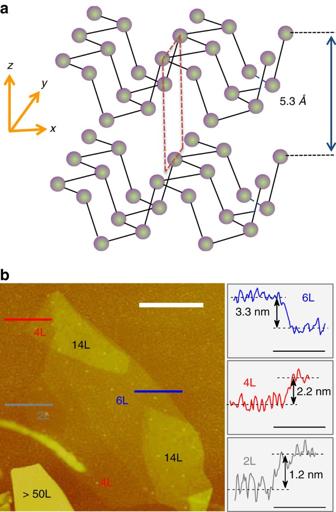Figure 1: Characterization of the thickness of black phosphorus. (a) Layered crystal structure of black phosphorus, showing the relative positioning of two adjacent puckered sheets with linked phosphorus atoms. The BP layer-to-layer spacing is around 5.3 Å. (b) Left: an AFM image of black phosphorus flakes. Estimated layer numbers are indicated. Scale bar (thick white): 2 μm. Right: line scans performed along the coloured lines shown in the left. Layer numbers from 2 to >50 are identified based on their thickness. Scale bar (grey): 1 μm. Figure 1: Characterization of the thickness of black phosphorus. ( a ) Layered crystal structure of black phosphorus, showing the relative positioning of two adjacent puckered sheets with linked phosphorus atoms. The BP layer-to-layer spacing is around 5.3 Å. ( b ) Left: an AFM image of black phosphorus flakes. Estimated layer numbers are indicated. Scale bar (thick white): 2 μm. Right: line scans performed along the coloured lines shown in the left. Layer numbers from 2 to >50 are identified based on their thickness. Scale bar (grey): 1 μm. Full size image In our experiments, multilayer BP was first exfoliated using the standard mechanical cleavage method from a bulk BP crystal and then deposited on a silicon substrate with 300-nm silicon dioxide. A typical atomic force microscope (AFM) image of thin-film BP is shown in Fig. 1b . Using a layer-to-layer spacing of 0.53 nm [36] , we clearly identified BP with thicknesses down to around 1.2 nm, corresponding to two atomic layers of BP. However, these few-micrometre scale bilayer BP flakes are usually too small for optical and electronic experiments. In this work, we performed optical and electrical measurements on BP layers with a thickness varying from 2 to >30 nanometres (4–60 layers). Polarization-resolved infrared spectroscopy For BP films thicker than 8 nm, flakes with a lateral size in the tens of micrometre scale can be isolated, allowing for the determination of crystalline directions using infrared spectroscopy [41] , [42] . The lower right inset of Fig. 2a shows an optical image of a BP flake with a thickness of around 30 nm. We measured the polarization-resolved relative extinction spectrum (1− T / T 0 ) in infrared, where T and T 0 are the optical transmission through the BP and the substrate and the substrate only, respectively. 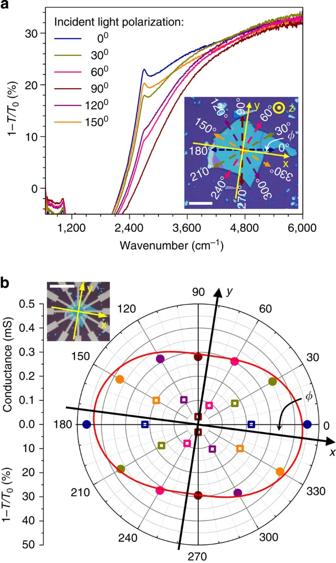Figure 2: Polarization-resolved infrared spectroscopy and angle-resolved DC conductivity of BP thin film. (a) Polarization-resolved infrared relative extinction spectra when light is polarized along the six directions as shown in the inset. Inset: an optical micrograph of a BP flake with a thickness of around 30 nm. Scale bar: 20 μm. (b) DC conductivity and IR relative extinction measured along the same six directions on this BP flake and plotted in polar coordinates. The angle-resolved DC conductance (solid dots) and the polarization-resolved relative extinction of the same flake at 2,700 cm−1(hollow squares) are shown on the same polar plot. Dots and squares of the same colour correspond to the directions indicated by the arrows in the inset ina. Inset: an optical image of this BP flake with 12 electrodes spaced at 30° apart. Scale bar: 50 μm. The crystalline orientation as determined by polarization-resolved IR measurements and angle-resolved DC conductance measurements match exactly. In botha,b,ϕis the angle between thexdirection and the 0° reference. Figure 2a denotes 1− T / T 0 measured on BP with the incident light from the z direction at six different linear polarization angles separated by 30 degrees, and indicated by the six arrowed lines with different colours in the inset. In this experiment, the 0° reference direction was selected arbitrarily. For all polarizations, the relative extinction shows a sharp increase at around 2,400 cm −1 , indicating a band gap of around 0.3 eV, which agrees very well with the previously reported BP band gap at the z symmetry point [36] . Since the optical conductivity of BP peaks in the x direction at the band edge [36] , by rotating the linear polarizer in finer steps, the angle between the x direction and the blue arrow (0° in Fig. 2a ) is determined to be −8°. The anisotropy in the optical conductivity arises from the directional dependence of the interband transition matrix elements in anisotropic BP bands [36] , [43] . Figure 2: Polarization-resolved infrared spectroscopy and angle-resolved DC conductivity of BP thin film. ( a ) Polarization-resolved infrared relative extinction spectra when light is polarized along the six directions as shown in the inset. Inset: an optical micrograph of a BP flake with a thickness of around 30 nm. Scale bar: 20 μm. ( b ) DC conductivity and IR relative extinction measured along the same six directions on this BP flake and plotted in polar coordinates. The angle-resolved DC conductance (solid dots) and the polarization-resolved relative extinction of the same flake at 2,700 cm −1 (hollow squares) are shown on the same polar plot. Dots and squares of the same colour correspond to the directions indicated by the arrows in the inset in a . Inset: an optical image of this BP flake with 12 electrodes spaced at 30° apart. Scale bar: 50 μm. The crystalline orientation as determined by polarization-resolved IR measurements and angle-resolved DC conductance measurements match exactly. In both a , b , ϕ is the angle between the x direction and the 0° reference. Full size image Angle-resolved DC conductance We also independently determined the x- and y directions of the BP thin film using an angle-resolved DC conductance measurement. In this experiment, 12 electrodes (1 nm Ti/20 nm Pd/30 nm Au) were fabricated on the same flake spaced at an angle of 30° along the directions as shown in the inset of Fig. 2b , which are along the same directions indicated by the coloured lines in Fig. 2a . Here we use the same 0° reference as that in the polarization-resolved infrared spectroscopy measurement in Fig. 2a . We performed these DC conductance measurements by applying an electric field across each pair of diagonally positioned electrodes separated by 22 μm at 180° apart and the results are plotted in Fig. 2b in polar coordinates. Measurements on each pair of electrodes lead to two data points in Fig. 2b separated by 180° for positive and negative bias, respectively. The directional dependence of the low-field conductivity in an anisotropic material can be described by the equation: σ θ = σ x cos 2 ( θ − ϕ )+ σ y sin 2 ( θ − ϕ ). The resulting calculated conductance fits nicely to the measurement data (red solid curve in Fig. 2b ). σ x and σ y refer to the conductivity of BP along the x - and y directions, respectively. θ is the angle, with respect to the 0° reference direction, along which both the electric field is applied and the conductance is measured. σ θ is the conductivity along the θ direction. ϕ is the angle between the x -direction and the 0° reference. ϕ =−8° gives the best fit for this sample ( Fig. 2b ), which agrees perfectly with the value obtained using infrared spectroscopy. Here, the x - and y directions correspond, respectively, to the high and low mobility directions, as shown in Fig. 1 . From the fitted curve, the ratio σ x / σ y is extracted to be around 1.5, corresponding to a ratio of the mobility along the x - and y directions μ x / μ y =1.5. Owing to the current spreading, this simple approach probably leads to an underestimation of the mobility anisotropy, as confirmed by the Hall measurement presented in the later part of this work. Polarization-resolved Raman scattering We further performed polarization-resolved Raman scattering measurements on the same BP flake discussed in the previous two sections with linearly polarized laser excitation incident from the z direction. This experimental configuration ( z in, z out) is the most relevant for layered BP thin films. The crystalline orientation of this single-crystal flake has already been identified using IR and DC conductivity experiments in the previous sections. The Raman scattering results for laser excitation light polarizations along the x , D and y directions are plotted in Fig. 3 . Here, the D direction is along the 45 ° direction to both the x and y directions within the x–y plane. We observe three Raman peaks in thin film BP at around 470, 440 and 365 cm −1 , corresponding to the , B 2g and modes, regardless of the polarization, which agrees well with previous observations in bulk BP crystals [44] . These sharp modes correspond to the unique orthorhombic crystalline phosphorus structure, confirming that the material studied in this work is indeed orthorhombic BP. Three other Raman active modes are not observed here because of the selection rules in this particular experimental configuration ( z in, z out). For all three different polarizations, we did not observe measurable peak position variations as the polarization changes. However, the relative intensity of these three peaks does change significantly with polarization direction. For example, as show in Fig. 3 , the B 2g mode clearly peaks when incident light is polarized along the D- direction because its intensity is determined only by the off-diagonal polarizability tensor α xy , which is maximized at 45° polarization [45] . The relatively intensity of the and modes varies significantly when the polarization changes. For both A g modes, the Raman scattering intensity is determined by both the diagonal and off-diagonal elements of the polarizability tensor and detailed theoretical investigations are needed to account for these variations. For BP films down to 3 nm, we also observed the same polarization dependence in the relative intensity of the , B 2g and modes, but again we did not observe any significant frequency shift in these three modes. While a more detailed discussion and modelling of the ( z in, z out) polarization-resolved Raman spectroscopy results and their dependence on the thin film thickness is not the focus of this paper, the polarization-resolved Raman measurements presented here offer another method for determining the crystalline directions of the BP thin film crystals. 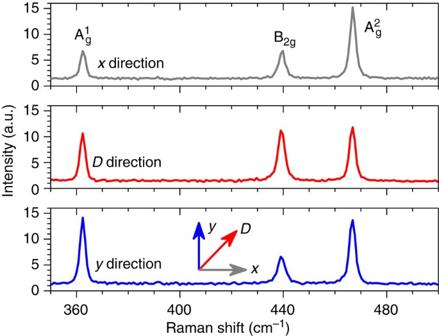Figure 3: Polarization-resolved Raman scattering. Polarization-resolved Raman spectra of a BP layered thin film with 532-nm linearly polarized laser excitation incident in thezdirection. Raman spectra with excitation laser polarization alongx- (grey),D- (red) andydirections (blue) are shown. TheDdirection is along 45° angle relative to thex- andydirections, as shown in the bottom panel. All spectra show, B2gandmodes. The peak positions do not change as the excitation light polarization varies. However, the relative intensities of these three modes change significantly with incident light polarization. The polarization-resolved Raman spectra can be used to identify the crystalline orientation of BP thin films, which is especially useful for relatively small flakes due to the small laser spot size (~1–2 μm). Figure 3: Polarization-resolved Raman scattering. Polarization-resolved Raman spectra of a BP layered thin film with 532-nm linearly polarized laser excitation incident in the z direction. Raman spectra with excitation laser polarization along x - (grey), D - (red) and y directions (blue) are shown. The D direction is along 45° angle relative to the x - and y directions, as shown in the bottom panel. All spectra show , B 2g and modes. The peak positions do not change as the excitation light polarization varies. However, the relative intensities of these three modes change significantly with incident light polarization. The polarization-resolved Raman spectra can be used to identify the crystalline orientation of BP thin films, which is especially useful for relatively small flakes due to the small laser spot size (~1–2 μm). Full size image Angle-resolved Hall mobility Using the infrared spectroscopy method described above, we first identified the crystalline directions in the BP thin films with a thickness of 8 and 15 nm. Standard Hall bars were fabricated on these thin films and the mobilities were measured in both the x - and y directions from 10 K to room temperature, as shown in Fig. 4 . For the 15 nm sample, the mobility along the x direction exceeds 600 cm 2 V −1 s −1 at room temperature and is above 1,000 cm 2 V −1 s −1 at 120 K. For the 8 nm sample, the mobility along the x direction exceeds 400 cm 2 V −1 s −1 at room temperature and is above 600 cm 2 V −1 s −1 at 120 K. The hole carrier density is kept at 6.7 × 10 12 cm −2 in all the measurements above. For both thicknesses, the Hall mobility along the x direction is about 1.8 times as large as that in the y direction, representing an anisotropy slightly smaller than that in bulk BP [36] but slightly larger than that extracted from the DC conductance measurement in Fig. 2b . Thicker BP consistently shows a higher mobility, indicating the impact of the substrate on the scattering of the carriers in BP thin films [46] . In bulk BP crystals, hole mobility values above 1,100 and 50,000 cm 2 V −1 s −1 along the x direction were previously reported at 300 and 30 K, respectively [36] . As a result, future improvement in BP thin film material quality is likely to result in much enhanced mobilities. The temperature dependence of the carrier mobility in BP shows a characteristic behaviour found in other layered materials. The initial increase in carrier mobility from 10 to 100 K is most likely due to the dominating Coulomb scattering mechanism [47] , [48] . As the temperature further increases, the mobility decreases due to phonon scattering following the power law relation ~ T − γ , with γ close to 0.5. This power law dependence is apparently weaker than in other 2D materials such as graphene and TMDCs [49] . Further theoretical and experimental lines of work are needed to clarify the temperature dependence of the mobility. 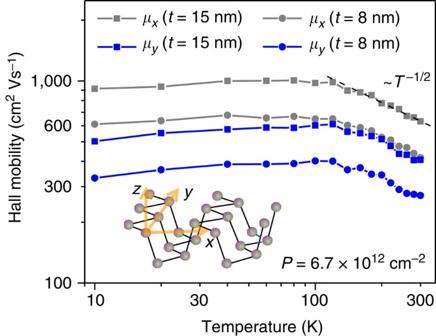Figure 4: Angle-resolved Hall mobility. Hall mobilities measured at a constant hole doping concentration of 6.7 × 1012cm−2along thex(μx) andy(μy) directions for BP thin films with a thickness of 8 and 15 nm, respectively.μxis about 1.8 times as large asμyand thicker films consistently show larger mobility than that of thinner films. Inset: schematic view of a single layer BP showing the crystalline directions. Figure 4: Angle-resolved Hall mobility. Hall mobilities measured at a constant hole doping concentration of 6.7 × 10 12 cm −2 along the x ( μ x ) and y ( μ y ) directions for BP thin films with a thickness of 8 and 15 nm, respectively. μ x is about 1.8 times as large as μ y and thicker films consistently show larger mobility than that of thinner films. Inset: schematic view of a single layer BP showing the crystalline directions. Full size image Transistors using x direction BP thin film as a channel material We also fabricated a series of transistors with a channel length of 1 μm using BP flakes with thicknesses varying from 2 to 15 nm. The transistor channels were intentionally designed along the x direction, as shown in the inset of Fig. 5b , which was determined using either infrared spectroscopy or Raman scattering as discussed above. 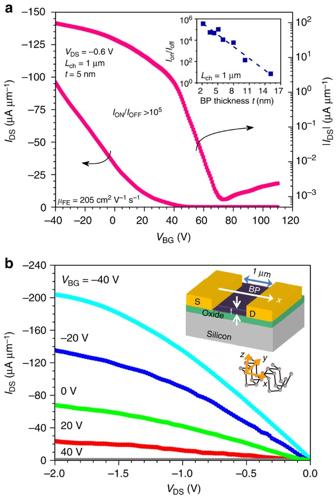Figure 5: Black phosphorus field-effect transistors along thexdirection. (a) Transfer characteristics of a field-effect transistor with a channel lengthLchof 1 μm using a BP thin film of around 5-nm thick.IDSandVBGare the source-drain current and back gate bias, respectively. The left and right axes represent linear and logarithmic scales, respectively. Inset: on–off current ratio as a function of BP thickness. (b) Output characteristics of the same transistor showing current saturation.VDSis the drain-source bias. All the transistors have channel lengths of 1 μm. Inset: a schematic view of the transistor. Thex-direction is indicated by the arrow. The black phosphorus crystalline directions (x,y, andz) are shown below the transistor schematic. Figure 5a,b denotes the transfer and output characteristics of a BP transistor at room temperature with a thickness of around 5 nm. An on–off current ratio exceeding 10 5 is achieved. In addition, plotted in Fig. 5a are the transfer characteristics on a linear scale, from which a field-effect mobility of 205 cm 2 V −1 s −1 is inferred using , where I DS is the source-drain current, V BG is the back gate bias, V DS is the source-drain bias, C ox is the gate capacitance, W is the width of the transistor and L is the channel length. Here, we emphasize that the field-effect mobility may be strongly affected by the traps in the device and the intrinsic band mobility can be much higher than 205 cm 2 V −1 s −1 , as shown in MoS 2 transistors [50] . Compared with graphene transistors, the BP devices consistently show much improved current saturation behaviour as shown in Fig. 5b . Finally, we plot the scaling of the on–off current ratio as a function of the BP thickness in the inset of Fig. 5a . For a BP thickness of 8 nm, the transistor on–off current ratio is 10 4 and the field-effect mobility is 300 cm 2 V −1 s −1 . For a BP thickness of around 2 nm, the on–off current ratio is as high as 5 × 10 5 . The field-effect mobility of this BP transistor is around 50 cm 2 V −1 s −1 , probably due to the greatly enhanced scattering by the substrate. However, we want to emphasize that this field-effect mobility may not represent the true carrier mobility because of traps and contact resistance [50] . The much improved transistor performance as compared with graphene indicates that the BP transistors can overcome the major shortcomings of graphene transistors in terms of on–off current ratio and current saturation. Combined with a much higher mobility than TMDCs, BP devices have great potential for applications in thin film radio-frequency electronics and logic circuits. Finally, as shown in Fig. 5a , the charge neutrality is achieved at a gate bias of around 70 V, corresponding to a hole doping of around 5 × 10 12 cm −2 . The exact origin of the doping is not clear and can be due to the adsorbates and contamination, and they may also adversely affect the carrier mobility. The intrinsic carrier mobility and doping mechanisms are important future research topics. Figure 5: Black phosphorus field-effect transistors along the x direction. ( a ) Transfer characteristics of a field-effect transistor with a channel length L ch of 1 μm using a BP thin film of around 5-nm thick. I DS and V BG are the source-drain current and back gate bias, respectively. The left and right axes represent linear and logarithmic scales, respectively. Inset: on–off current ratio as a function of BP thickness. ( b ) Output characteristics of the same transistor showing current saturation. V DS is the drain-source bias. All the transistors have channel lengths of 1 μm. Inset: a schematic view of the transistor. The x -direction is indicated by the arrow. The black phosphorus crystalline directions ( x , y , and z ) are shown below the transistor schematic. Full size image In summary, we have reintroduced BP as an anisotropic material with a narrow bandgap and a high carrier mobility to the layered-material family. It bridges the energy gap between the semimetallic graphene and various large bandgap TMDCs, making BP thin films an ideal candidate for various near and mid-infrared optoelectronic applications, such as photodetectors and modulators. Moreover, because of its relatively high carrier mobility and good current saturation properties, thin-film BP has great potential to surpass graphene as a novel and more favourable material for high performance RF and logic applications in thin-film electronics. Most importantly, its unique angle-dependent properties allow a new degree of freedom for designing conceptually new optoelectronic and electronic devices, which are not possible using other 2D materials. For example, BP is a natural material for developing mid-infrared polarizers and polarization sensors, while its angle-dependent optical conductivity may allow the construction of plasmonic devices where the surface plasmon polariton frequency will have a strong directional dependence on the wave vector. Owing to its anisotropic nature, BP also offers advantages for building better transistors along its light effective-mass ( x ) direction. The low effective mass can help to obtain high-performance quasi-ballistic transistors at advanced technology nodes where the channel lengths are comparable to the mean free path of carriers by achieving higher low-field mobility, overshoot velocity and on-state current [25] , [26] , [27] . These are just a few of the promising applications of BP that we have identified, while an entire family of novel device concepts that can utilize the angle-dependent properties of this intriguing material awaits our exploration. During the preparation of this manuscript, we became aware of two experimental works studying the electronic properties of BP on arXiv.org (arXiv:1401.4117v1 and arXiv:1401.4133v1). During the revision process, these two manuscripts and one additional experimental work were published [51] , [52] , [53] . Transistor and Hall bar fabrication The fabrication of our devices starts with the exfoliation of BP thin films from bulk BP crystals on 300 nm SiO 2 on a Si substrate, which has pre-patterned alignment grids, using the micromechanical cleavage technique. The thickness of the SiO 2 was selected to provide the optimal optical contrast for locating BP flakes relative to the alignment grids and for roughly estimating their thicknesses. The number of BP layers was then confirmed using AFM based on the sample thickness. The next step was to pattern the resist layer for metallization using a Vistec 100 kV electron-beam lithography system based on poly (methyl methacrylate) (950k MW PMMA). PMMA A3 was spun on wafer at a speed of 3,000 r.p.m. and was then bakes at 175° for 3 min. The dose for exposure is 1,100 μC cm −2 . Development was performed in 1:3 MIBK: IPA (Methyl isobutyl ketone: Isopropanol). We then evaporated 1 nm Ti/20 nm Pd/30 nm Au followed by lift-off in acetone to form the contacts. AFM and Raman spectroscopy AFM for identifying the thin-film thickness was performed on a Digital Instruments/Veeco Dimension 3000 system. Polarization-resolved Raman spectroscopy was performed using a 532-nm Nd:YAG laser in the LabRAM ARAMIS system. We used a × 100 microscope objective and the power incident on BP was kept below 500 μW to avoid sample damage. Infrared spectroscopy Infrared spectroscopy was performed in the 800–6,000 cm −1 range using a Bruker Optics Fourier Transfer Infrared spectrometer (Vertex 70) integrated with a Hyperion 2000 microscope system. Incident light polarization was achieved using an infrared polarizer. Electrical characterization All electrical characterizations were performed using an Agilent 4155C semiconductor parameter analyser and a Lakeshore cryogenic probe station with micromanipulation probes. How to cite this article: Xia, F. et al. Rediscovering black phosphorus as an anisotropic layered material for optoelectronics and electronics. Nat. Commun. 5:4458 doi: 10.1038/ncomms5458 (2014).